Coordinated DNA dynamics during the human telomerase catalytic cycle The human telomerase reverse transcriptase (hTERT) utilizes a template within the integral RNA subunit (hTR) to direct extension of telomeres. Telomerase exhibits repeat addition processivity (RAP) and must therefore translocate the nascent DNA product into a new RNA:DNA hybrid register to prime each round of telomere repeat synthesis. Here, we use single-molecule FRET and nuclease protection assays to monitor telomere DNA structure and dynamics during the telomerase catalytic cycle. DNA translocation during RAP proceeds through a previously uncharacterized kinetic substep during which the 3′-end of the DNA substrate base pairs downstream within the hTR template. The rate constant for DNA primer realignment reveals this step is not rate limiting for RAP, suggesting a second slow conformational change repositions the RNA:DNA hybrid into the telomerase active site and drives the extrusion of the 5′-end of the DNA primer out of the enzyme complex. Specialized nucleoprotein structures called telomeres protect the ends of eukaryotic chromosomes from aberrant recognition and processing by DNA damage repair proteins [1] , [2] . The inability of conventional replication machinery to generate a complete copy of telomere DNA results in gradual telomere shortening with each round of cell division and limits the proliferative capacity of cells [3] . However, in rapidly dividing cell types, including the majority of human cancers, the enzymatic activity of telomerase maintains telomere length by adding short telomere DNA repeats (GGTTAG in humans) to chromosome ends [4] , [5] , [6] . The function of the telomerase ribonucleoprotein complex relies on contributions from multiple evolutionarily conserved domains within the telomerase reverse transcriptase (hTERT) protein and RNA (hTR) subunits [7] , [8] . Telomerase recognizes the 3′-end of single-stranded telomere DNA via Watson–Crick base pair interactions with the hTR template, forming an RNA:DNA hybrid, which is then extended by hTERT to generate a complete telomere DNA repeat [8] , [9] . Synthesis of a single telomere DNA repeat by telomerase proceeds through a mechanism similar to other DNA polymerases and reverse transcriptases [10] . In contrast, telomerase displays a unique repeat addition processivity (RAP) activity, during which the nascent telomere RNA:DNA hybrid dissociates and realigns downstream in the hTR template, permitting the addition of multiple telomere repeats to the growing DNA chain before dissociation ( Fig. 1a ) [11] , [12] , [13] . 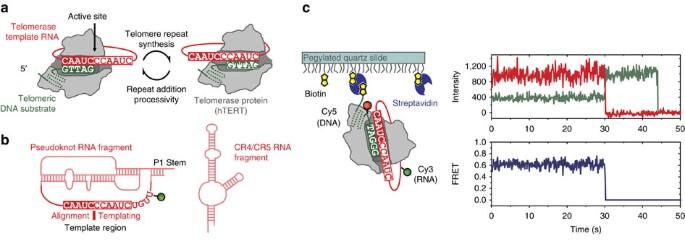Figure 1: A single-molecule FRET assay for monitoring telomerase–DNA interactions. (a) A model for telomere DNA repeat synthesis and RAP during the telomerase catalytic cycle. The precise location of the primer outside of the template hybrid is not well characterized and is therefore represented by a dashed line to denote an arbitrary path for the primer as it exits complex. (b) Cartoon schematics of the two hTR fragments used in telomerase reconstitutions. The pseudoknot fragment is shown with a U42-Cy3 modification. (c) (left) Schematic illustration of experimental geometry during smFRET telomerase binding experiments using total internal reflection fluorescence microscopy. (right) A representative single-molecule trajectory of U42-Cy3-labelled telomerase bound to the 18GGG/T13-Cy5 primer. (top) Raw donor Cy3 (green) and acceptor Cy5 (red) dye intensities and (bottom) calculated FRET values are plotted as a function of time. The sudden drop in the dye intensity traces represents irreversible photobleaching of the FRET dyes. Figure 1: A single-molecule FRET assay for monitoring telomerase–DNA interactions. ( a ) A model for telomere DNA repeat synthesis and RAP during the telomerase catalytic cycle. The precise location of the primer outside of the template hybrid is not well characterized and is therefore represented by a dashed line to denote an arbitrary path for the primer as it exits complex. ( b ) Cartoon schematics of the two hTR fragments used in telomerase reconstitutions. The pseudoknot fragment is shown with a U42-Cy3 modification. ( c ) (left) Schematic illustration of experimental geometry during smFRET telomerase binding experiments using total internal reflection fluorescence microscopy. (right) A representative single-molecule trajectory of U42-Cy3-labelled telomerase bound to the 18GGG/T13-Cy5 primer. (top) Raw donor Cy3 (green) and acceptor Cy5 (red) dye intensities and (bottom) calculated FRET values are plotted as a function of time. The sudden drop in the dye intensity traces represents irreversible photobleaching of the FRET dyes. Full size image Telomere DNA primer length and 5′-sequence composition are critical determinants of RAP, indicating that binding interactions apart from the RNA:DNA hybrid contribute to telomerase function [6] , [14] , [15] . DNA crosslinking experiments have identified specific points of contact between the telomerase essential N-terminal (TEN) domain of hTERT and telomere DNA primers [16] , [17] . In addition, hTERT harbours a conserved RT primer grip motif, which mediates interactions with the RNA:DNA hybrid and is crucial for proper RAP [18] , [19] , [20] . Thus, discrete points of telomerase–DNA contact prevent enzyme dissociation during the complex DNA handling required for RAP [21] ; however, the precise details of how the DNA binding properties of telomerase are modulated during multiple rounds of telomere repeat synthesis remain unknown. Single-molecule approaches have been used to interrogate conformational rearrangements of numerous polymerase–nucleic acid complexes, providing novel insight into how template and product strands are dynamically bound and restructured during both DNA and RNA synthesis [22] , [23] . For example, single-molecule Förster resonance energy transfer (smFRET) revealed a DNA-scrunching mechanism for RNA polymerase during early stages of transcriptional initiation [24] , mapped the exit path of nascent messenger RNA out of eukaryotic RNA polymerase II [25] and revealed the nucleic acid binding orientation dynamics of the HIV reverse transcriptase [26] , [27] . Here, we have used smFRET paired together with nuclease protection mapping experiments to characterize the structural dynamics and kinetic sub-states of telomere DNA substrates during telomerase catalysis. Our results reveal that single-stranded telomere DNA primers exhibit a compact conformation during early stages of repeat synthesis. On completion of a telomere repeat, the 3′-end of the nascent DNA dynamically samples a new base pairing register in the downstream region of the hTR template. Interestingly, kinetic characterization of this primer realignment substep indicates that a subsequent rearrangement of the telomerase complex must be rate limiting for complete translocation during RAP. We further characterized DNA rearrangements during the rate-limiting step of RAP using biochemical footprinting experiments, which suggested that repositioning of the realigned RNA:DNA hybrid in the active site is accompanied by the extrusion of the 5′-end of the DNA substrate out of the enzyme complex. Taken together, our results support a model for telomerase RAP, during which coordinated DNA movements serve to both prime the synthesis of subsequent telomere repeats as well as render the 5′-end of the DNA substrate accessible to trans -acting proteins such as the POT1-TPP1 processivity factor [28] . A single-molecule assay for human telomerase–DNA interactions To analyse telomerase–DNA interactions by smFRET, enzyme complexes were reconstituted in vitro using a previously reported two-piece RNA system [29] (Pseudoknot nt 32–195 and CR4/CR5 nt 239-328), harbouring a site-specific Cy3 (donor) modification at position U42, located 5′ of the RNA template ( Fig. 1b and Supplementary Fig. 1 ). Total internal reflection fluorescence microscopy was used to measure the distance-dependent energy transfer between the Cy3 dye within hTR and a Cy5 (acceptor) label within the telomere DNA primer, reporting on the relative positions of the DNA primer and the hTR subunit within the complex ( Fig. 1c ). We recently reported a similar experimental design for the T. thermophila telomerase enzyme [30] , [31] ; however, the capacity of human telomerase to bind certain DNA primer sequences with extremely high affinity ( t 1/2 >20 h (ref. 32 )) permits purification of the active telomerase fraction [33] and greatly facilitates the single-molecule experiments in the present study. Importantly, all FRET modified telomerase enzymes and telomere DNA primers supported near wild-type levels of activity and processivity as measured by direct DNA primer extension assays ( Supplementary Fig. 2 ). For our initial measurements, we utilized an 18 nucleotide (nt) telomere DNA primer terminating in ‘GGG’ at the 3′-end (18GGG). The primer was site-specifically modified with an internal Cy5 dye covalently coupled to a thymine at position 13 (from the 5′ end) in the DNA primer (18GGG/T13, Fig. 2a ). This DNA sequence permutation promotes a high-affinity telomerase–DNA interaction [32] and permits efficient primer-dependent surface immobilization of telomerase complexes onto the streptavidin-coated microscope slide using a 5′ biotin moiety ( Fig. 1c and Supplementary Fig. 3 ). Single-molecule FRET trajectories revealed a stable FRET=0.59 state and exhibited single-step photobleaching of the FRET dyes ( Fig. 1c and Fig. 2b ), characteristic of a single telomerase complex bound to a DNA primer. Thus, human telomerase functions as a monomer under the conditions of our assay, consistent with previous single-molecule studies of in vitro -reconstituted human telomerase enzymes [34] , but in contrast to several reports that have demonstrated human telomerase can exist as a functional dimer when reconstituted in vivo [35] , [36] . 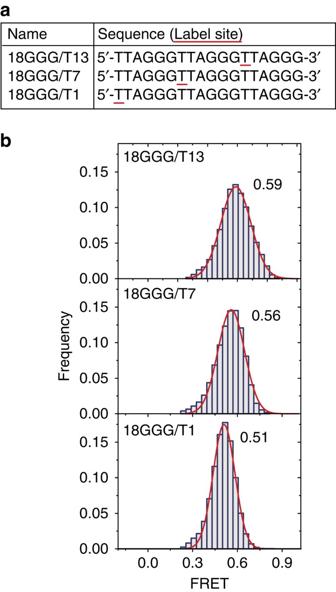Figure 2: Telomere DNA substrate is compacted within the telomerase complex. FRET histograms for the 5′-biotinylated 18GGG/T13-Cy5 (top), 18GGG/T7-Cy5 (middle), and 18GGG/T1-Cy5 (bottom) DNA primers. Histograms were fit with Gaussian functions (red lines) to determine the indicated centres of each FRET distribution. All histograms in the figure are constructed from at least 2000 individual molecules. Figure 2: Telomere DNA substrate is compacted within the telomerase complex. FRET histograms for the 5′-biotinylated 18GGG/T13-Cy5 (top), 18GGG/T7-Cy5 (middle), and 18GGG/T1-Cy5 (bottom) DNA primers. Histograms were fit with Gaussian functions (red lines) to determine the indicated centres of each FRET distribution. All histograms in the figure are constructed from at least 2000 individual molecules. Full size image We next tested whether the surface-immobilized telomerase–DNA complexes were competent to catalyse DNA synthesis. At time zero, a smFRET histogram constructed from several 100 telomerase–DNA complexes displayed a single dominant FRET population centred at FRET=0.59 ( Fig. 2b and Supplementary Fig. 4a ), consistent with the individual FRET traces ( Fig. 1b ). Addition of dNTPs to the sample chamber promotes a time-dependent shift of the FRET distribution to lower FRET values, which ultimately centres at FRET=0.07 after a 60-min incubation ( Supplementary Fig. 4b,c ). Since the donor Cy3 dye is incorporated into the telomerase enzyme, the shift to lower FRET values cannot be explained by enzyme dissociation over time. Moreover, smFRET histograms constructed from telomerase–DNA complexes incubated for 60 min in the absence of dNTPs, or with a catalytically dead telomerase mutant (D868A) [37] , show no deviation from the initial FRET distribution ( Supplementary Fig. 4d,e ). These data indicate that the majority of the surface-immobilized telomerase–DNA complexes in our experiments are competent to bind and catalytically extend a DNA primer. Telomerase-catalyzed DNA synthesis manifests itself as a gradual shift of the smFRET distribution to an extremely low FRET state, suggesting that the DNA primer, and possibly telomerase itself, undergoes considerable rearrangements during multiple rounds of processive telomere repeat synthesis. DNA rearrangements during telomere repeat synthesis To further explore the conformation of the DNA bound within the telomerase–DNA complex, we next measured the smFRET distributions for a series of 18 nt ‘GGG’ terminating primers labelled with Cy5 at three different positions (T13, T7, and T1; Fig. 2b ). Again, all modified DNA primers supported near wild-type level activity and processivity in DNA primer extension assays ( Supplementary Fig. 2b ). The smFRET histograms constructed from data collected with 18GGG/T13, 18GGG/T7 and 18GGG/T1 all yielded unimodal distributions, which were well-fit by single Gaussian functions centred at FRET=0.59, 0.56 and 0.51, respectively ( Fig. 2b ). These data suggest that the entire 18 nt DNA primer assumes a compact conformation within the core telomerase complex. We next set out to analyse how the conformation of the DNA changes with the stepwise addition of dNTPs during telomere DNA repeat synthesis. To this end, surface-immobilized telomerase–DNA complexes were incubated for 30 min with specific combinations of dNTPs and ddNTPs to terminate the reaction at precisely controlled stages of repeat synthesis beginning with the high-affinity 18GGG/T13 primer sequence ( Supplementary Fig. 2b , lanes 8–11). To simplify interpretation of these smFRET measurements, we first tested whether the position of the U42-Cy3 label site within the hTR subunit is stationary throughout the repeat synthesis reaction. Doubly labelled hTR molecules harbouring U42-Cy3 and U29-Cy5 modifications were reconstituted into a catalytically active telomerase complex ( Supplementary Figs 1 and 2 lane 6). Notably, the immobilization of doubly labelled telomerase complexes onto the microscope slide was DNA primer dependent, as evidenced by the background level of telomerase complexes observed in the absence of biotinylated DNA primer ( Supplementary Fig. 3 ). At each successive stage of telomere repeat synthesis, the FRET value measured between hTR positions U29 and U42 remained constant ( Fig. 3a ). This result is somewhat surprising in light of a similar experiment performed on the Tetrahymena telomerase enzyme, which suggested that regions of RNA flanking the template undergo conformational rearrangements during the telomere repeat synthesis reaction [30] . Thus, the observation that hTR position U42 remains stationary with respect to U29 (P1 stem) during telomere repeat synthesis may reflect a distinct structural property of the human telomerase enzyme (see Discussion). 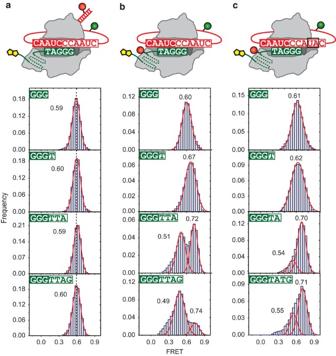Figure 3: DNA conformational changes induced by completion of telomere DNA repeat synthesis. (a) FRET distributions constructed with doubly labelled telomerase enzyme harbouring hTR U29-Cy5 (P1 stem) and U42-Cy3 dyes initially bound to 5′ biotinylated 18GGG primer. FRET histograms at each indicated step of the repeat synthesis reaction are shown and fit with single Gaussian functions (red lines) centred at FRET ~0.6 (dotted line). Initial 3′ DNA sequence is highlighted in green and nascent DNA sequence is highlighted in white. (b) FRET distributions constructed from U42-Cy3-labelled telomerase enzyme initially bound to 18GGG/T13-Cy5 DNA primer and extended to each indicated step of the repeat synthesis reaction are shown. Data were fit with either one or two Gaussian functions (red lines) to determine the indicated centres of each FRET distribution. (c) FRET distributions constructed from U42-Cy3-labelled telomerase enzyme harbouring the template mutations UA47-48AU, initially bound to the 18GGG/T13-Cy5 primer and extended to each indicated step of the repeat synthesis reaction are shown. Data were fit with either one or two Gaussian functions (red lines) to determine the indicated centres of each FRET distribution. All histograms in the figure are constructed from at least 500 individual molecules. Figure 3: DNA conformational changes induced by completion of telomere DNA repeat synthesis. ( a ) FRET distributions constructed with doubly labelled telomerase enzyme harbouring hTR U29-Cy5 (P1 stem) and U42-Cy3 dyes initially bound to 5′ biotinylated 18GGG primer. FRET histograms at each indicated step of the repeat synthesis reaction are shown and fit with single Gaussian functions (red lines) centred at FRET ~0.6 (dotted line). Initial 3′ DNA sequence is highlighted in green and nascent DNA sequence is highlighted in white. ( b ) FRET distributions constructed from U42-Cy3-labelled telomerase enzyme initially bound to 18GGG/T13-Cy5 DNA primer and extended to each indicated step of the repeat synthesis reaction are shown. Data were fit with either one or two Gaussian functions (red lines) to determine the indicated centres of each FRET distribution. ( c ) FRET distributions constructed from U42-Cy3-labelled telomerase enzyme harbouring the template mutations UA47-48AU, initially bound to the 18GGG/T13-Cy5 primer and extended to each indicated step of the repeat synthesis reaction are shown. Data were fit with either one or two Gaussian functions (red lines) to determine the indicated centres of each FRET distribution. All histograms in the figure are constructed from at least 500 individual molecules. Full size image We next measured FRET between the U42-Cy3 and the DNA primer with the T13-Cy5 modification. The centre of the initial FRET=0.59 peak gradually increases, until the synthesized repeat terminates with ‘TTA’ or ‘TAG’, at which point a new significantly lower FRET=0.49 state is observed ( Fig. 3b ). Analysis of individual smFRET trajectories revealed a dynamic interconversion between the FRET=0.74 and FRET=0.48 states for 18GGG/T13 primers extended to the complete telomere DNA repeat sequence ( Fig. 4a ). Single-molecule FRET traces were fit using a hidden Markov model to yield idealized FRET trajectories [38] , and the individual times spent in each FRET state ( τ were binned into dwell-time distributions ( Fig. 4b ). Both distributions were well-fit by single exponential decay functions, yielding mean dwell times < τ > FRET=0.48 =38±8.1 s and < τ > FRET=0.74 =10±1.6 s, corresponding to the rate constants k 0.48–>0.74 =0.026±0.0059, s −1 and k 0.74–>0.48 =0.098±0.015 s −1 . Notably, the value we measure for k 0.74–>0.48 is ~100-fold faster than previously reported estimates for the rate constant governing RAP measured by ensemble primer extension assays under similar experimental conditions [39] . 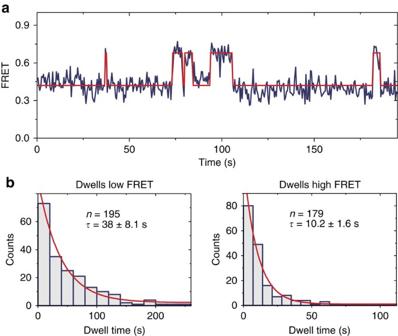Figure 4: Kinetic analysis of DNA primer dynamics induced on completion of a telomere DNA repeat. (a), A representative single-molecule trace of a telomerase complex that has completed synthesis of a single telomere DNA repeat exhibiting multistate FRET dynamics. The calculated FRET ratio is plotted as a function of time (blue line). Data were fit using the HaMMy software package to generate idealized FRET trajectories (red line). (b), Dwell-time histograms of the times spent in either the low FRET=0.48 state (left) or high FRET=0.74 state (right) are plotted and fit with single exponential decay functions yielding average dwell times <τ> of 38±8.1 and 10±1.6 s for the low FRET and high FRET states, respectively. These mean dwell times correspond to the rate constantsk0.48−>0.74=0.0026±0.0059 andk0.74−>0.48=0.098±0.015 s−1. The sample sizes represent the number of individual transitions used in the analysis and error estimates represent s.e.m. Figure 4: Kinetic analysis of DNA primer dynamics induced on completion of a telomere DNA repeat. ( a ), A representative single-molecule trace of a telomerase complex that has completed synthesis of a single telomere DNA repeat exhibiting multistate FRET dynamics. The calculated FRET ratio is plotted as a function of time (blue line). Data were fit using the HaMMy software package to generate idealized FRET trajectories (red line). ( b ), Dwell-time histograms of the times spent in either the low FRET=0.48 state (left) or high FRET=0.74 state (right) are plotted and fit with single exponential decay functions yielding average dwell times < τ > of 38±8.1 and 10±1.6 s for the low FRET and high FRET states, respectively. These mean dwell times correspond to the rate constants k 0.48−>0.74 =0.0026±0.0059 and k 0.74−>0.48 =0.098±0.015 s −1 . The sample sizes represent the number of individual transitions used in the analysis and error estimates represent s.e.m. Full size image To further characterize the novel FRET=0.48 conformation, we next utilized a mutant hTR (UA47-48AU) containing the altered template sequence, 3′-AAUCCCA UA C-5′. This mutant enzyme can bind the 18GGG/T13 primer with wild-type affinity and extend to the end of the first telomere DNA repeat [40] . However, the mismatches introduced into the nascent DNA sequence disrupt base pairing with the downstream region of the hTR template and substantially abrogate RAP ( Supplementary Fig. 2b , lane 7), as previously reported [40] . When the UA47-48AU enzyme was analysed in the smFRET assay, we again observed an increase in the initial FRET=0.61 state as seen with the wild-type enzyme, but the stability of the low FRET conformation at the end of repeat synthesis was significantly reduced ( Fig. 3c ). These results provide evidence that the stability of the FRET=0.48 intermediate relies on correct base pairing between the nascent DNA product and the downstream region of the hTR template, and that formation of this previously uncharacterized translocation intermediate is not the rate-limiting step during RAP. Telomere DNA movements during RAP To analyse DNA rearrangements required for the complete RAP cycle, we employed a single round translocation assay [39] to measure the DNA conformations during the initial binding, telomere DNA repeat synthesis and RAP phases of the telomerase catalytic cycle ( Fig. 5 ). For these experiments, we used a 21 nt DNA primer with a T7-Cy5 modification terminating with the sequence ‘TTA’ (21TTA/T7, see Supplementary Table 1 ). On initial binding, we observed a bimodal FRET distribution consistent with our previous experiments performed with the 18GGG/T13 primer (compare Figs 3b and 5a). Addition of a single ddGTP completes the first telomere repeat and further stabilizes the low FRET=0.41 translocation intermediate, again consistent with our previous results (compare Figs 3b ). The presence of both dGTP and ddTTP should promote a single round of RAP during which telomerase completes the first telomere repeat, translocates and then continues to add nucleotides until synthesis is terminated by incorporation of a ddTTP. However, RAP is not highly efficient in the absence of the trans -acting cofactors POT1-TPP1 ( Supplementary Fig. 5a ) [28] , [39] . Therefore, we established a technique to enrich for telomerase enzymes that have successfully completed one round of RAP by exploiting the difference in binding affinity for telomere DNA primers terminating in ‘TAG’ and ‘GGT’ [32] . Telomerase enzyme was prebound to the 5′ biotinylated 21TTA/T7 primer in a centrifuge tube, and then activated to extend the primer by addition of dGTP and ddTTP in the presence of excess 18GGG chase primer ( Supplementary Fig. 5b ). In this way, complexes that successfully completed a RAP cycle converted the low-affinity 21TTA/T7 primer to a high-affinity 25GGT/T7 primer and are selectively immobilized on the glass slide for smFRET measurements ( Supplementary Fig. 5c ). These single round RAP complexes yielded a unimodal FRET distribution centred at FRET=0.49 ( Fig. 5c ), a value that is consistent with the conformation of the DNA primer established with the 18GGG series of primers (compare Fig. 5c with Fig. 2b 18GGG/T1). Taken together, these results suggest that the translocation process during RAP is comprised of at least two distinct steps: (i) a rapid realignment of the 3′-end of the complete telomere DNA repeat with the downstream region of the hTR template ( Fig. 5b ), and (ii) a second, rate-limiting conformational rearrangement during which the realigned RNA:DNA hybrid is repositioned in the hTERT active site to prime the next round of repeat synthesis. 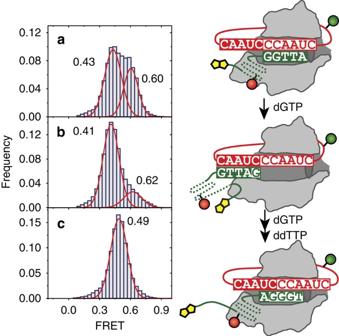Figure 5: DNA conformational changes during RAP. (a) FRET histogram constructed from U42-Cy3-labelled telomerase bound to 21TTA/T7-Cy5 DNA primer. (b) FRET histogram constructed from U42-Cy3-labelled telomerase initially bound to 21TTA/L2, surface immobilized on the microscope slide and incubated in 200 μM ddGTP to complete the synthesis of a single telomere DNA repeat. (c) FRET histogram for U42-Cy3-labelled telomerase enzyme initially bound to 21TTA/T7-Cy5, incubated in 200 μM dGTP and ddTTP to permit one round of RAP in the presence of excess high-affinity chase 18GGG primer, followed by surface immobilization for FRET measurements as described in the main text andSupplementary Fig. 5. FRET distributions in all panels were fit with either single or double Gaussian functions (red lines) to determine the indicated position of each FRET distribution. All histograms in the figure are constructed from at least 700 individual molecules. Figure 5: DNA conformational changes during RAP. ( a ) FRET histogram constructed from U42-Cy3-labelled telomerase bound to 21TTA/T7-Cy5 DNA primer. ( b ) FRET histogram constructed from U42-Cy3-labelled telomerase initially bound to 21TTA/L2, surface immobilized on the microscope slide and incubated in 200 μM ddGTP to complete the synthesis of a single telomere DNA repeat. ( c ) FRET histogram for U42-Cy3-labelled telomerase enzyme initially bound to 21TTA/T7-Cy5, incubated in 200 μM dGTP and ddTTP to permit one round of RAP in the presence of excess high-affinity chase 18GGG primer, followed by surface immobilization for FRET measurements as described in the main text and Supplementary Fig. 5 . FRET distributions in all panels were fit with either single or double Gaussian functions (red lines) to determine the indicated position of each FRET distribution. All histograms in the figure are constructed from at least 700 individual molecules. Full size image 5′ DNA primer extrusion during RAP The similarity of the observed FRET conformations for the 18GGG/T1 ( Fig. 2 ) and the 25GGT/T7 ( Fig. 5c ) primers raised the intriguing possibility that during RAP, repositioning of the RNA:DNA hybrid is coupled with 5′ DNA extrusion out of the enzyme complex. While suggestive, our smFRET results alone are not sufficient to firmly support this model for coordinated movements of the 3′ and 5′ ends of the DNA primer. Therefore, we used a recently established footprinting assay that exploits the 5′→3′ nuclease activity of ExoVII to probe how much telomere DNA is protected when bound to telomerase [41] . For these experiments, all telomere DNA primers possessed at least three copies of natural telomere DNA sequence and a 10 nt 5′-polyT extension. The use of a polyT sequence to extend the length of the primer was strategically chosen to avoid complications introduced by the formation of a stable intramolecular G-quadruplex in the DNA primer [42] , [43] . In addition, primers were added at ~200-fold greater concentrations than telomerase to minimize the possibility of multiple enzymes binding a single DNA substrate in our assays, thereby simplifying interpretation of the footprinting data. Telomere DNA primers prebound to telomerase were activated for extension by the addition of dGTP [α 32 P] and ddTTP for the indicated period of time, followed by a 5-min treatment with ExoVII to digest exposed 5′-single-stranded DNA ( Fig. 6a ). ExoVII treatment was limited to 5 min to ensure that the signal obtained was derived from stable telomerase–DNA complexes, rather than probing DNA that dissociated from the telomerase enzyme. Importantly, since telomerase incorporates radiolabeled dGTP into the cold DNA primer, all bands observed on the gel represent products of active telomerase complexes. 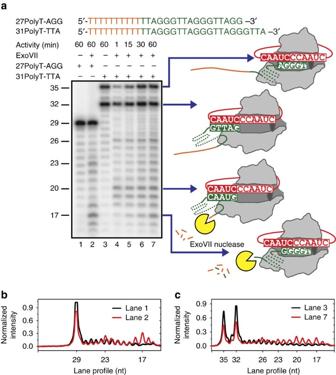Figure 6: Exonuclease VII digestion reveals extrusion of 5′ DNA during RAP. (a) Autoradiogram of a 12% denaturing PAGE gel resolving the products of telomerase-catalyzed primer extension of the indicated telomere DNA primers (27PolyT-AGG or 31PolyT-TTA). Telomerase extension products of the 27PolyT-AGG primer in the presence of 200 μM dGTP [α32P] and ddTTP, untreated (Lane 1) or treated (Lane 2) with ExoVII. (Lane 3) Telomerase extension products of the 31PolyT-TTA primer in the presence of dGTP [α32P] and ddTTP. (Lanes 4–7) Time-course of telomerase extension of 31PolyT-TTA in the presence of dGTP [α32P] and ddTTP followed by ExoVII treatment. (b) Lane profiles for 27PolyT-AGG extended primer untreated (Lane 1, black) and ExoVII treated (Lane 2, red). (c) Lane profiles for 31PolyT-TTA extended primer untreated (Lane 3, black) and ExoVII treated (Lane 7, red). All lane profiles have been normalized by the total intensity of the lane. Figure 6: Exonuclease VII digestion reveals extrusion of 5′ DNA during RAP. ( a ) Autoradiogram of a 12% denaturing PAGE gel resolving the products of telomerase-catalyzed primer extension of the indicated telomere DNA primers (27PolyT-AGG or 31PolyT-TTA). Telomerase extension products of the 27PolyT-AGG primer in the presence of 200 μM dGTP [α 32 P] and ddTTP, untreated (Lane 1) or treated (Lane 2) with ExoVII. (Lane 3) Telomerase extension products of the 31PolyT-TTA primer in the presence of dGTP [α 32 P] and ddTTP. (Lanes 4–7) Time-course of telomerase extension of 31PolyT-TTA in the presence of dGTP [α 32 P] and ddTTP followed by ExoVII treatment. ( b ) Lane profiles for 27PolyT-AGG extended primer untreated (Lane 1, black) and ExoVII treated (Lane 2, red). ( c ) Lane profiles for 31PolyT-TTA extended primer untreated (Lane 3, black) and ExoVII treated (Lane 7, red). All lane profiles have been normalized by the total intensity of the lane. Full size image We first used a 27 nt primer terminating with the sequence ‘AGG’ (27PolyT-AGG, Fig. 6a ), which under the conditions of our experiments will incorporate a single dGTP and then terminate with ddTTP to yield a single 29 nt product ( Fig. 6a , lane 1). We observed a small amount of shorter non-specific degradation products not present in the untreated DNA primer sample ( Supplementary Fig. 6a ), which is likely a result of a minor nuclease contaminant. When DNA in this complex is partially digested with ExoVII, we observe two regions of protection centred about a predominant 17 nt band and a second 23 nt band ( Fig. 6a , lane 2 and Fig. 6b ). Interestingly, the length of the 23 nt protected fragment suggests the 5′-end of the DNA primer can adopt two conformations that maintain a 6 nt spacing. To address the question of what happens to the 5′-end of the DNA during a single round of RAP, we used a 31 nt primer terminating with the sequence ‘TTA’ (31PolyT-TTA, Fig. 6a ), which is compatible with single round translocation experiments. In the absence of ExoVII, extension of this primer produces two predominant products: one 32 nt band corresponding to the addition of one dGTP which completes synthesis of the full telomere repeat, and a second 35 nt band representing successful RAP and extension of the next telomere repeat until termination by ddTTP incorporation ( Fig. 6a , lane 3). At early stages of a reaction time course with the 31PolyT-TTA primer, the 32 nt product accumulates, and when treated with ExoVII, gives rise to protected fragments centred about a 20 and 26 nt ( Fig. 6a , lane 4). These products precisely correspond to the 5′-protection pattern we observed for the 27PolyT-AGG primer, suggesting the 5′ most contact is maintained throughout telomere repeat synthesis. As the reaction proceeds, the amount of the 35 nt RAP product increases, and when these complexes are treated with ExoVII, two additional protected fragments are observed centred about 17 and 23 nt ( Fig. 6a , lane 7 and Fig. 6c ). The accumulation of these new cleavage products correlates with accumulation of the 35 nt extension product ( Supplementary Fig. 6b ), supporting the notion that these shorter ExoVII fragments are derived from digestion of primers that have undergone RAP. As described above, RAP is not highly efficient under the conditions of our assay, and therefore ExoVII products generated for the single round translocation reactions represent a superimposition of products derived from complexes that have stalled at the end of telomere repeat synthesis and those that have undergone a single RAP cycle. To deconvolute these cleavage patterns, we performed a control experiment with a 32 nt primer terminating with ‘TAG’ (32 PolyT-TAG) to enrich for the 35 nt RAP product, which when treated with ExoVII exclusively produced the protected fragments centred about 17 and 23 nt ( Supplementary Fig. 6c ). These results provide direct physical evidence that extrusion of the 5′ end of the DNA out of the enzyme is coupled to completion of a RAP cycle. We present a model for the dynamic handling of DNA during telomerase catalysis that integrates our results together with existing biochemical data ( Fig. 7 ). In this model, telomerase initially binds its telomere DNA substrate via a combination of base pairing interactions with the template region of the integral hTR subunit, together with distinct contacts in the 5′-region of the DNA substrate (i). Once bound, a single telomere DNA repeat is rapidly synthesized. Interestingly, our smFRET approach revealed that on completion of the telomere DNA repeat synthesis reaction, a dynamic equilibrium exists, wherein the 3′-end of the nascent DNA primer transiently samples different alignment registers of the hTR template (ii). Our novel single-molecule assay provided the first direct quantitative characterization of this obligatory step during telomerase RAP. Existing models for telomerase catalysis suggest the denaturation of the nascent RNA:DNA hybrid is the kinetically slow step during RAP [12] , [44] , [45] , [46] ; however, our data demonstrate that this step is fast compared with the overall rate for RAP that has been reported in the literature [39] . Therefore, to reconcile our smFRET results with ensemble assays for RAP, we propose a subsequent rate-limiting conformational rearrangement of the telomerase complex serves to reposition the realigned RNA:DNA hybrid into the hTERT active site to prime the subsequent round of repeat addition (iv). During this slow conformational rearrangement, the 5′ end of the DNA primer is extruded out of the enzyme complex. This model is consistent with the recent report by Qi et al . that inferred rebinding of the RNA:DNA duplex in the hTERT active site may be required during RAP from trans template complementation experiments. 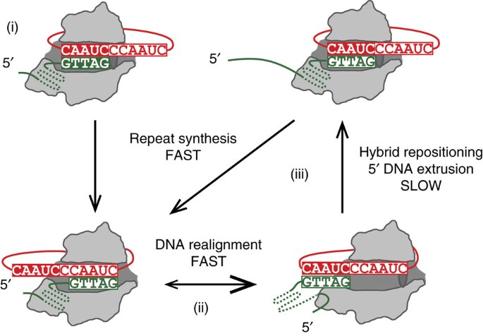Figure 7: Model for DNA conformational rearrangements during telomerase catalytic cycle. (i) Telomerase initially binds a telomere DNA substrate through RNA:DNA hybrid interactions with the template and additional 5′-DNA contacts. Rapid synthesis of a complete telomere DNA repeat extends the RNA:DNA hybrid to the template boundary, at which point a dynamic equilibrium of DNA primer states exists (ii), favoring the formation of a realigned RNA:DNA hybrid. (iii) In a second, rate-limiting, step of RAP, the realigned RNA:DNA hybrid is repositioned in the telomerase active site and the 5′-end of the DNA primer is extruded from the enzyme complex. Figure 7: Model for DNA conformational rearrangements during telomerase catalytic cycle. (i) Telomerase initially binds a telomere DNA substrate through RNA:DNA hybrid interactions with the template and additional 5′-DNA contacts. Rapid synthesis of a complete telomere DNA repeat extends the RNA:DNA hybrid to the template boundary, at which point a dynamic equilibrium of DNA primer states exists (ii), favoring the formation of a realigned RNA:DNA hybrid. (iii) In a second, rate-limiting, step of RAP, the realigned RNA:DNA hybrid is repositioned in the telomerase active site and the 5′-end of the DNA primer is extruded from the enzyme complex. Full size image A recent smFRET analysis of Tetrahymena telomerase revealed the RNA template and/or flanking regions undergo conformational rearrangements during telomere repeat synthesis [30] . These previous experiments would appear to contradict the present finding that hTR-U42 is stationary throughout the repeat synthesis reaction. However, it is possible that the template region, rather than the 5′ flanking sequence, is the major source of structural compliance within telomerase RNA during telomere repeat synthesis. An alternative, but not mutually exclusive, explanation for the observed smFRET results may relate to differences in the mechanism of template boundary definition for the human and Tetrahymena telomerase enzymes. This notion is in accordance with recent biochemical evidence from Wu et al ., [41] which demonstrated that template definition in human telomerase is an intrinsic property of RNA:DNA hybrid recognition, rather than being externally defined by adjacent protein–RNA contacts as described for the Tetrahymena system [48] . The telomerase enzyme used for the experiments in the present work was reconstituted using the well-established rabbit reticulocyte lysate system [37] , [49] . This telomerase reconstitution approach has been reported to yield monomeric enzyme complexes [34] , consistent with our single-molecule FRET trajectories which exhibit single-step photobleaching behaviour. In contrast, human telomerase reconstituted in human cell lines can produce a dimeric telomerase complex [33] , though the structural basis for dimerization remains unknown. Despite this difference in oligomerization state, a recent study showed that in vitro - and in vivo -reconstituted telomerase complexes exhibit similar functional properties with respect to DNA primer handling [41] . In addition, a recent analysis of many disease-associated alleles of telomerase components led to the conclusion that the individual monomers within the dimeric telomerase complex act independently [36] . However, a separate study that analysed the catalytic properties of telomerase complexes harbouring one active and one catalytically dead subunit found that a non-functional mutant telomerase monomer can act in a dominant-negative fashion and abrogate the catalytic activity of the wild-type monomer [35] . While the source of this discrepancy remains unknown, the majority of available experimental evidence supports the notion that the DNA handling properties characterized for the monomeric telomerase complexes used in the present study will generally apply to the individual monomers within a telomerase dimer. The regulated extrusion of the DNA primer out of the telomerase complex has direct implications for the molecular mechanism of the trans -acting telomerase cofactor POT1/TPP1, which dramatically increases the rate and efficiency of RAP [28] , [39] . Previous experiments utilizing a mutant hTR template that produced a telomere DNA repeat sequence incapable of binding POT1/TPP1 demonstrated that a DNA primer harbouring a single 5′ wild-type POT1/TPP1 binding site could be processively extended, suggesting that POT1/TPP1 may remain stably associated with telomerase during multiple rounds of RAP [39] . Subsequently, the so-called ‘TEL patch’ was shown to mediate the interaction of POT1/TPP1 with telomerase [50] , and single-molecule experiments revealed that POT1/TPP1 can dynamically slide along telomere DNA primers [51] . Our results suggest that six nucleotides of DNA are extruded from the telomerase complex with each round of RAP, an amount of telomere DNA that is smaller than the established ten nucleotide binding site size of POT1 (refs 28 , 39 ). Thus, as DNA is released with each round of RAP, the POT1/TPP1 dimer associated with telomerase would be expected to dynamically slide along the growing DNA chain before another POT1/TPP1 complex can bind. Preparation of RNAs In vitro transcription In vitro reconstitution of telomerase enzyme was performed using the established two RNA fragment system in which the essential RNA pseudoknot domain and the CR4/CR5 domain are added in trans [52] , [53] . Unlabelled CR4/CR5 RNA (hTR 239-328) was generated by in vitro transcription using T7 RNAP and polyacrylamide gel electrophoresis (PAGE) purified. Site-specific RNA labelling within the RNA pseudoknot domain was achieved using DNA-splinted RNA ligation techniques as described previously [54] . Unlabelled fragments of the RNA pseudoknot domain (hTR 63–195 and hTR 63–201) were prepared by in vitro transcription using T7 RNAP and purified using a 6% denaturing PAGE gel. Subsequently, the RNA was phosphatase (CIP, NEB) treated to remove the 5′ triphosphate, phenol/chloroform extracted to remove CIP, T4 PNK (NEB) treated to add a 5′ monophosphate, phenol/chloroform extracted to remove PNK and PAGE purified to remove excess nucleotide. Both enzymatic reactions were carried out using NEB specifications. Synthetic, dye-labelled RNA fragments Synthetic RNA fragments were purchased from Dharmacon containing internal aminoallyl uridines (5-N-U) used for dye labelling reactions. Specific RNA sequences are listed in Supplementary Table 1 . RNAs were generally processed as previously described [54] with the following exceptions. All ethanol precipitation steps were replaced by purification over a GE PD-midiTRAP G25 column. RNA in each fraction was identified by NanoDrop or by eye once a dye label was present. The fractions were pooled and evaporated to dryness using a vacuum centrifuge set at 45 °C. If a 5′ phosphate was required for ligation, the dye-labelled oligos were phosphorylated by PNK treatment, followed by phenol/chloroform extraction. Ligation of RNA fragments Modifications of the previously reported procedure [55] included addition of 1 U μl −1 RNasin and carrying out the ligation overnight at 30 °C. The DNA splints for each RNA ligation are listed in Supplementary Table 1 . Note for the doubly RNA labelled construct, the U29 and U42 fragments were ligated and purified before ligation with the in vitro transcribed fragment. Preparation of telomerase enzyme Telomerase reconstitution Telomerase reconstitution was performed using the TnT Quick Coupled Transcription/Translation system (Promega) [55] . For every 100 μl of TnT Quick mix, 2 μg of pNFLAG-hTERT was added. RNAs were then added to the reaction mixture where dye-labelled RNAs were added to a final concentration of 0.1 μM, whereas all unlabelled RNAs were added to 1 μM. The reconstitution mixture was held at 30 °C for 3 h. Telomerase purification Directly after reconstitution, telomerase enzymes were purified using an N-terminal FLAG tag on hTERT. To pull down the enzyme, Sigma Anti-FLAG M2-agarose bead slurry was used at 50 μl bead slurry per 200 μl lysate. The beads were first washed four times with wash buffer (50 mM Tris HCl pH 8.3, 3 mM MgCl 2 , 2 mM DTT, 1 mM spermidine, 100 mM KCl), spinning at 2350, r.c.f., 4 °C, for 1 min between washes. The beads were blocked while being agitated in 750 μl blocking buffer (50 mM Tris HCl pH 8.3, 3 mM MgCl 2 , 2 mM DTT, 1 mM spermidine, 0.5 mg ml −1 BSA, 0.05 mg ml −1 glycogen, 0.1 mg ml −1 yeast tRNA) for 15 min at 4 °C. After spinning the beads at 2,350 r.c.f., 4 °C, for 1 min the supernatant was discarded. The blocking step was repeated and then the beads were added to the lysate. The beads were agitated at 4 °C for 2 h allowing the prepared enzyme to associate with the anti-FLAG beads. The mixture was spun at 2,350 r.c.f., 4 °C, for 1 min and the supernatant was discarded. The beads were then washed with 750 μl of wash buffer and spun at 2,350 r.c.f., 4 °C, for 1 min. This process was repeated four times to remove residual lysate. To elute the enzyme, 60 μl of elution buffer (50 mM Tris HCl pH 8.3, 3 mM MgCl 2 , 1 mM spermidine, 0.5 mg ml −1 BSA, 10% glycerol, 0.75 mg ml −1 3 × FLAG peptide) was added for every 200 μl of lysate and the slurry was incubated at 4 °C for one hour. Beads were removed by centrifugation filtration using a Nanosep MF 0.45 μm filter. From this solution, 10-μl aliquots were prepared, flash frozen in liquid nitrogen and stored at −70 °C until use. DNA primer extension assays Activity assays were performed using 5 μl of purified enzyme diluted to a final volume of 10 μl in 1 × activity buffer. Each reaction maintained a final concentration of 1 μM primer substrate, 250 μM dATP, 250 μM dTTP, 1 μM α 32 P-dGTP (PerkinElmer BLU514Z500UC), and 1 × activity buffer (50 mM Tris HCl pH 8.3, 3 mM MgCl 2 , 2 mM DTT, 1 mM spermidine). The reactions were initiated by addition of dNTPs and incubated at 30 °C for 90 min unless noted otherwise. Reactions monitoring stepwise addition of dNTPs to a DNA primer were performed for 30 min in the presence of a combination of 250 μM dNTPs plus the appropriate chain terminating ddNTPs at 250 μM ( Supplementary Fig. 2 , lanes 8–11). Reactions were terminated by addition of 90 μl stopping buffer (10 mM Tris HCl pH 7.5, 1 mM EDTA, 0.1% w/v SDS). The reactions were mixed vigorously with 100 μl of phenol to remove protein components followed by a 10 min spin at 15,000 r.c.f. The aqueous layer was further extracted with 100 μl of chloroform and spun at 15,000 r.c.f. for 2 min. After isolation of the aqueous phase, the radiolabeled DNA was precipitated and then separated on a 12% denaturing PAGE gel (19:1 crosslinking ratio). The gel was dried, exposed on a phosphorimager screen overnight and scanned using a Typhoon scanner. Quantification of the bands was accomplished by using SAFA v11b [56] . Preparation of dot blot oligo probe The 24 nt DNA probe ( Supplementary Table 1 ) hybridizes to pseudoknot nt 130–153. 10 pmol probe oligo was 5′ 32 P labelled using 10 μl γ 32 P-ATP (PerkinElmer BLU002Z250UC). The reaction was carried out in 1 × PNK Buffer (NEB) at a total volume of 20 μl with 10 U of PNK (NEB). The probe was purified using two sequential Centri-Spin 10 columns following the manufacturer’s protocol. Dot blot quantification of enzyme concentration To quantify the concentration of telomerase we determined the concentration of telomerase pseudoknot RNA in the Immuno-precipitated enzyme solution. First a serial dilution of in vitro transcribed pseudoknot RNA was made as an internal standard (10 fmol μl −1 , 5 fmol μl −1 , 1 fmol μl −1 and 0.5 fmol μl −1 ). For each of the standard RNA solutions and the reconstituted enzymes, 1 μl of sample was made up with 9 μl of formamide buffer (90% formamide, 0.1% bromophenol blue, 0.1% xylene cyanol, 1 × TBE). The samples were heated at 70 °C for 5 min and the put on ice. After cooling, the samples were applied to a Hybond N+ membrane (GE Life Sciences RPN119B). The samples were air dried and then UV-crosslinked to the membrane using a Stratagene Stratalinker 1800 set to the ‘Auto-crosslink’ programme. The membrane was prehybridized at 55 °C in 10 ml of Church buffer (1% BSA Fraction V, 1 mM EDTA pH 7.5, 500 mM Na 2 HPO 4 , pH 7.2, 7% SDS) for 30 min. A total of 1 × 10 6 c.p.m. of 32 P labelled dot blot oligo probe was then added to the hybridization buffer and incubated overnight at 55 °C. The membrane was washed with 150 ml of 0.1 × SSC/0.1 × SDS three times to remove excess probe. After air-drying, the membrane was exposed on phosphorimager screen and imaged using a Typhoon scanner. Quantification of the blot intensities was accomplished using ImageJ 1.45S. Single-molecule experiments Slide preparation Quartz slides (Finkenbeiner Inc.) were cleaned and pegylated using the following protocol [57] . The slides were boiled in water to remove parafilm and coverslips from previous experiments. The slides were then scrubbed with alconox (Alconox Inc.), rinsed and placed into a solution containing 10% alconox. After sonication for 20 min, the slides were rinsed and placed in water and sonicated for 5 min. Slides were then sonicated in acetone for 15 min. The slides were directly transferred into 1 M KOH and sonicated for 20 min. After thorough rinsing, the slides surfaces were flame dried and cleaned using a butane torch (BernzOmatic). While the slides were cooling, a silanizing solution containing 100 ml of methanol, 5 ml of glacial acetic acid and 1 ml of N-(2-aminoethyl)-3-aminopropyltrimethoxysilane (UCT) was prepared. The cooled slides were placed in the solution, sonicated for 1 min and allowed to stand in solution at room temperature for at least 20 min. While incubating slides, 200 mg of mPEG-Succinimidyl Valerate MW 5,000 (Laysan Bio, Inc.), was resuspended in 400 μl of 0.1 M NaHCO 3 . Also 2 mg of Biotin-PEG-Succinimidyl Valerate MW 5,000 (Laysan Bio, Inc.) was resuspended in 200 μl of 0.1 M NaHCO 3 . After rinsing the slides with dH 2 O and drying with nitrogen, the solutions were mixed and applied to each slide surface (150 μl per slide). A coverslip was used to cover the solution and the slides incubated overnight at room temperature in a humidor box. The following day, channels were assembled using Paramfilm as a spacer on the pegylated quartz slides and plasma-cleaned coverslips were used as the second chamber face [55] . Incubation and molecule deposition To prepare the slides for molecule deposition, the channels were incubated with 60 μl of 10 mg ml −1 BSA (NEB) for 20 min. The slide was then washed with 100 μl of T50 (10 mM Tris HCl pH8, 50 mM NaCl) and then incubated with 60 μl of 0.2 mg ml −1 streptavidin in T50 for 5 min. After coating the slide with streptavidin, the excess protein was washed away with 500 μl of T50. While preparing the slide, 10 μl of purified enzyme was incubated with 1 μl of 10 nM biotinylated primer for 1 h at room temperature. After incubation, the molecules were diluted with 20 μl of imaging buffer (50 mM Tris HCl pH 8.3, 3 mM MgCl 2 , 1 mM spermidine, 0.5 mg ml −1 BSA, 4% glucose) and flowed over the slide surface. The number of molecules on the surface was observed in real time to reach the desired density for smFRET measurements. Once telomerase molecules were deposited on the surface, the stable complexes were retained and imaged after multiple buffer exchanges. Imaging of the FRET-labelled enzymes required an oxygen-scavenging system and a triplet state quencher to increase dye lifetime. Imaging buffer did not substantially impact telomerase activity ( Supplementary Fig. 2 , lanes 14 and 15). The buffer was saturated with Trolox (triplet state quencher), passed through a 0.22-μm filtration unit and brought to pH 8.3. Once ready for imaging, the solution was brought to 2 μg ml −1 catalase and 1 mg ml −1 glucose oxidase. The pH was found to be stable for more than 30 min with these conditions (data not shown). DNA extension by surface-immobilized telomerase complexes After telomerase–DNA complexes were immobilized on the microscope slide, the indicated dNTPs or combination of dNTPs+ddNTPs were added as described in the text at a concentration of 200 μM. The reaction was allowed to proceed for 30 min before washing the channel with imaging buffer and collecting single-molecule FRET data. Microscope setup Data were collected using a custom built prism-type microscope, allowing hundreds of molecules to be studied in parallel [54] . Cy3 donor dyes were directly excited with a 532 nm laser (Laserglow). Depending on the proximity of Cy5 acceptor dye to the donor dye, a variable degree of energy transfer will occur from the excited donor dye to the acceptor dye. Due to this FRET process, both dyes are capable of fluorescing and emit at distinct wavelengths. Emitted fluorescence was split into separate donor and acceptor channels using dichroic mirrors, and imaged on an EM-CCD camera (Andor Ixon). Data acquisition and analysis Imaging fields containing 30–250 molecules were imaged using a 100 ms integration time for fast timescale traces and histograms and 500 ms integration time for slow timescale traces. Individual traces were parsed out using custom written IDL software where they were corrected for background and dye-crosstalk signal (software available on request). The individual traces were then filtered in MATLAB using a thresholding analysis where molecules containing no acceptor dye were discarded. FRET intensities were then calculated using the equation I A / ( I A + γI D ) where I A is the acceptor intensity, I D is the donor intensity and γ is the gamma correction factor. The gamma correction factor was determined as described [57] for a subset of ~100 molecules, averaged and applied to the entire dataset. The first 5 s of individual FRET traces were then binned into FRET histograms. Zero peaks resulting from premature photobleaching were subsequently removed by either subtraction of a Gaussian fit from the data set or deletion of the data entirely where applicable. The center of the FRET distributions were determined by a non-linear Gaussian fitting algorithm and reported next to each fit. HaMMy and dwell-time analysis Hidden Markov Modelling (HaMMy, http://bio.physics.illinois.edu/HaMMy.html ) was used for identification and fitting of FRET states. Fits were brought into MATLAB where the idealized FRET traces generated by HaMMy were parsed into individual dwell times and binned in an array that was used to generate dwell-time histograms. Dwell-time histograms were fit with a single exponential decay function yielding a characteristic relaxation time, τ , which is equivalent to the inverse of the rate constant. Exonuclease VII experiments Initially, 1 μM primer was mixed with 10 μl of purified telomerase and incubated for 30 min at RT to promote binding. A master mixture was made and added to the telomerase solution providing final conditions of activity buffer, 1 μM α32P-dGTP (Perkin Elmer BLU014Z500UC) and 200 μM ddTTP. In the case of Exonuclease VII digestion, telomerase activity reactions were allowed to proceed for the indicated length of time and 20 U of Exonuclease VII (Epicentre EN510250) was added and incubated at room temperature for 5 min. The reaction was quenched with 80 μl stopping buffer (10 mM Tris HCl pH 7.5, 1 mM EDTA, 0.1% w/v SDS). After phenol/chloroform extraction, the products were ethanol precipitated, resolved on a 12% denaturing PAGE gel (19:1 crosslinking ratio), and exposed on a phosphorimager screen overnight. Quantification of the bands was accomplished by using SAFA v11b [56] . The lane profiles seen in Fig. 6b,c and Supplementary Fig. 6b were generated by taking a cross section of each lane in ImageJ and normalizing the values to the total lane counts. How to cite this article: Parks, J. W. and Stone, M. D. Coordinated DNA dynamics during the human telomerase catalytic cycle. Nat. Commun. 5:4146 doi: 10.1038/ncomms5146 (2014).